IRF8 directs stress-induced autophagy in macrophages and promotes clearance ofListeria monocytogenes Autophagy, activated by many stresses, plays a critical role in innate immune responses. Here we show that interferon regulatory factor 8 (IRF8) is required for the expression of autophagy-related genes in dendritic cells. Furthermore in macrophages, IRF8 is induced by multiple autophagy-inducing stresses, including IFNγ and Toll-like receptor stimulation, bacterial infection, starvation and by macrophage colony-stimulating factor. IRF8 directly activates many genes involved in various steps of autophagy, promoting autophagosome formation and lysosomal fusion. Consequently, Irf8 −/− macrophages are deficient in autophagic activity, and excessively accumulate SQSTM1 and ubiquitin-bound proteins. We show that clearance of Listeria monocytogenes in macrophages requires IRF8-dependent activation of autophagy genes and subsequent autophagic capturing and degradation of Listeria antigens. These processes are defective in Irf8 −/− macrophages where uninhibited bacterial growth ensues. Together these data suggest that IRF8 is a major autophagy regulator in macrophages, essential for macrophage maturation, survival and innate immune responses. Autophagy is a catabolic process by which misfolded self-proteins and damaged organelles are captured and enzymatically degraded [1] , [2] . Autophagy is activated by a variety of stress signals such as starvation and inflammation [1] . In macrophages (MФs) and dendritic cells (DCs), autophagy is also triggered by inflammatory cytokines such as interferonγ (IFNγ), ligands for Toll-like receptors (TLRs) and other pathogen recognition receptors and is required for innate clearance of invading pathogens [3] , [4] , [5] , [6] . The absence of autophagy genes such as Atg5 and Atg7 impairs pathogen recognition activity, type I IFN production and increases susceptibility to pathogens, including Mycobacterium (M) tuberculosis and Listeria monocytogenes [7] , [8] , [9] , [10] . Recent studies indicate that autophagy is involved in M-CSF-induced differentiation of monocytes to MФs [11] , [12] . Autophagy follows a well-ordered sequence of events where the activation of ULK1 and Beclin1 leads to LC3 lipidation and autophagosome formation. Autophagosomes then fuse with lysosomes to allow the hydrolysis of captured materials. Autophagic degradation is linked to the ubiquitin conjugation pathway, as some ubiquitinated proteins are escorted to autolysosomes through ubiquitin adaptors such as SQSTM1 (p62) to allow proteasome independent degradation [10] , [13] , [14] . IFNγ-induced GTPases, such as IRGM1, are recruited to the autolysosomes and facilitate autophagic clearance of bacteria [15] . It is thought that autophagic activation and the subsequent elimination of captured molecules are directed by a mechanism that unifies and coordinates complex autophagic processes [1] . Although our understanding on this aspect of autophagy is limited, there are a few examples where autophagic events are joined together as a defined network: in these cases, transcription factors, such as TEFB and FOXO3 act as autophagy master regulators in a cell type- and signal-dependent manner [16] , [17] . Interferon regulatory factor 8 (IRF8) is a transcription factor that promotes the differentiation of MФs and DC subsets [18] , [19] . IRF8 is induced by IFNγ plus TLRs in MФs and stimulates genes important for host defense, including type I IFNs, promoting the production of reactive oxygen species and nitric oxide [20] , [21] . IRF8 is essential for innate resistance against intracellular bacteria, including M. tuberculosis , M. Bovis ( BCG ), Salmonella and Listeria, although underlying mechanisms have not been fully understood [22] , [23] , [24] , [25] , [26] . We show here that IRF8 is induced in MФs and DCs by diverse stresses that activate autophagy and stimulates transcription of many autophagy genes, thereby facilitating the entire autophagic processes. Accordingly, Irf8 −/− MФs are defective in various steps of autophagy induced by IFNγ/TLR stimulation, Listeria infection, starvation and macrophage colony-stimulating factor (M-CSF). As a result, ubiquitin-linked SQSTM1 accumulates in greater amounts in Irf8 −/− MФs than wild-type (WT) MФs. Further, infection by Listeria monocytogenes leads to a dramatically induced IRF8 that coincides with marked activation of multiple autophagy genes, which results in autophagic control of bacterial growth. Irf8 −/− MФs are, however, unable to activate autophagy genes and succumb to uninhibited Listeria growth. Transfer of the Irf8 gene into Irf8 −/− MФs partially rescues the expression of autophagy genes and autophagic activity in Listeria infected MФs. Together, IRF8 is an autophagy master regulator that acts in MΦs to meet diverse stresses. Microarray analyses reveal a role of IRF8 in autophagy Previous genome-wide studies reported that IRF8 regulates more than 1,500 genes in monocytes, MФs and B cells [21] , [27] , [28] . To gain genome-wide information on IRF8 in DCs, we performed microarray analyses with bone marrow (BM)-derived DCs from WT and Irf8 −/− mice on stimulation by TLR ligands, lipopolysaccharide (LPS) and CpG. With a cutoff line of >2 × with P ≤0.05 (identified by one-way analysis of variance), 326 and 713 genes were expressed higher in WT DCs than in Irf8 −/− DCs in untreated (UT) and TLR-stimulated DCs, respectively ( Fig. 1a , left), whereas the expressions of 350 and 648 genes were lower in WT DCs than in Irf8 −/− DCs ( Fig. 1a , right). Thus, IRF8 regulates many constitutive and TLR-stimulated genes in DCs either positively or negatively, as reported before for other cell types [21] , [27] , [28] . Gene ontology (GO) analysis of positively regulated genes showed significant enrichment for immune system processes, inflammatory responses, lysosome functions, while genes negatively regulated by IRF8 were enriched with cell cycle, cell division and DNA replication ( Supplementary Fig. 1a,b ). A large number of TLR-stimulated genes were upregulated by IRF8, consistent with previous reports that IRF8 is critical for TLR activation of DCs ( Supplementary Fig. 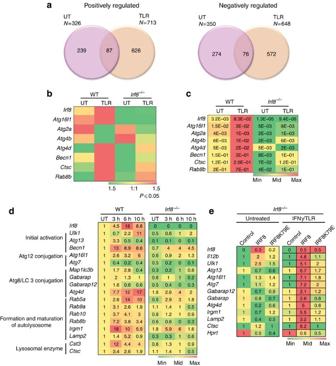Figure 1: Microarray analyses reveal a role of IRF8 in autophagy. (a) The Venn diagrams depict the number of genes positively and negatively regulated by IRF8 in UT DCs and those treated with TLR ligands for 6 h identified by microarray analysis. Overlapped regions represent the number of genes positively or negatively regulated both in UT and TLR-stimulated DCs. See GO classification inSupplementary Fig. 1a,b. (b) IRF8-dependent autophagy genes identified by microarray analysis. Differentially expressed genes were identified by one-way analysis of variance (P≤0.05 and fold change ≥2). Colour gradients indicate average signal intensities of genes in log2 scale. Normalization was performed by GeneChip Operating Software (GCOS) and Expression Console software’s relative to the UT. (c) qRT–PCR analysis of IRF8-dependent autophagy genes in DCs. WT andIrf8−/−DCs were stimulated with the TLR ligands for 6 h. The numbers represent transcript levels normalized bygapdhlevels. Data represent the average of three independent assays.P≤0.01, Student’st-test. (d) qRT–PCR analysis of IRF8-dependent autophagy genes in MΦs. WT andIrf8−/−MΦs were treated overnight with IFNγ and stimulated with TLR ligands for the indicated times. The number in each box represents transcript levels normalized by the value of UT WT cells. Values are the average of three independent assays.P≤0.01 (Student’st-test). See autophagy genes not affected by IRF8 inSupplementary Fig. 2. (e)Irf8−/−MФs were transduced with pMSCV retroviral vector containing WTIrf8or mutantIrf8(K79E), and stimulated with IFNγ/TLR for 8 h. Relative expression of indicated autophagy genes was detected by qRT–PCR. The numbers represent transcript levels normalized by those of cells transduced with empty vector.Irf8expression was normalized bygapdh. Values are the average of three experiments.P≤0.05 (Student’st-test).Il12bandHprtwere tested as controls. 1c and Supplementary Table 1 ) [18] , [20] , [29] . Eleven percent of those were found in the Interferome, confirming a functional link between IRF8- and IFN-related regulation ( http://interferome.org/ ) [30] ( Supplementary Fig. 1d ). Figure 1: Microarray analyses reveal a role of IRF8 in autophagy. ( a ) The Venn diagrams depict the number of genes positively and negatively regulated by IRF8 in UT DCs and those treated with TLR ligands for 6 h identified by microarray analysis. Overlapped regions represent the number of genes positively or negatively regulated both in UT and TLR-stimulated DCs. See GO classification in Supplementary Fig. 1a,b . ( b ) IRF8-dependent autophagy genes identified by microarray analysis. Differentially expressed genes were identified by one-way analysis of variance ( P ≤0.05 and fold change ≥2). Colour gradients indicate average signal intensities of genes in log2 scale. Normalization was performed by GeneChip Operating Software (GCOS) and Expression Console software’s relative to the UT. ( c ) qRT–PCR analysis of IRF8-dependent autophagy genes in DCs. WT and Irf8 −/− DCs were stimulated with the TLR ligands for 6 h. The numbers represent transcript levels normalized by gapdh levels. Data represent the average of three independent assays. P ≤0.01, Student’s t -test. ( d ) qRT–PCR analysis of IRF8-dependent autophagy genes in MΦs. WT and Irf8 −/− MΦs were treated overnight with IFNγ and stimulated with TLR ligands for the indicated times. The number in each box represents transcript levels normalized by the value of UT WT cells. Values are the average of three independent assays. P ≤0.01 (Student’s t -test). See autophagy genes not affected by IRF8 in Supplementary Fig. 2 . ( e ) Irf8 −/− MФs were transduced with pMSCV retroviral vector containing WT Irf8 or mutant Irf8 (K79E), and stimulated with IFNγ/TLR for 8 h. Relative expression of indicated autophagy genes was detected by qRT–PCR. The numbers represent transcript levels normalized by those of cells transduced with empty vector. Irf8 expression was normalized by gapdh . Values are the average of three experiments. P ≤0.05 (Student’s t -test). Il12b and Hprt were tested as controls. Full size image Inspection of IRF8-stimulated genes belonging to the category of immune system processes and lysosome functions ( Supplementary Fig. 1a ) revealed that a number of genes in the autophagy pathway are downregulated in Irf8 −/− DCs ( Fig. 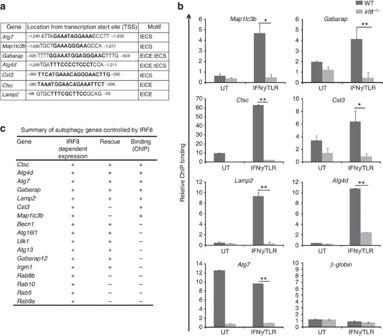Figure 2: IRF8 binds to the promoters of autophagy genes. (a) Consensus IRF8-binding motifs are shown in bold on indicated autophagy gene promoters. (b) IRF8 binding to the above motifs was detected by ChIP for WT andIrf8−/−MФs (UT or treated with IFNγ/TLR) normalized by normal IgG binding, and withβ-globinas a negative control. Values represent the average of five independent experiments. *P≤0.05 and **P≤0.01. (Student’st-test). (c) Summary of qRT-PCR analysis rescue experiment and ChIP assays. 1b and Supplementary Table 2 ). These genes, except for Atg2a , were induced after TLR, as confirmed by quantitative reverse transcription-PCR (qRT–PCR) analysis ( Fig. 1c ). Because IRF8 regulates shared sets of genes in DCs and MФs and autophagy has been extensively investigated in MФs, we hereafter studied the role of IRF8 in MФ autophagy. The expressions of 24 autophagy genes were first tested in BM-derived MФs from WT and Irf8 −/− mice stimulated with IFNγ overnight followed by TLR ligands, LPS and CpG: IFNγ and TLR ligands provide priming and triggering signals, respectively, which together boost autophagic activity in MФs [31] , [32] . Data in Fig. 1d showed that 17 autophagy genes were downregulated in Irf8 −/− MФs relative to WT MФs and that all but Atg7 were induced by IFNγ plus TLR (IFNγ/TLR) stimulation. Atg7 expression, which fell after stimulation, was also consistently lower in Irf8 −/− MФs than WT cells. These genes represent essentially all phases of autophagy (see Fig. 1d , left). As reported previously, IFNγ/TLR treatment also stimulated Irf8 expression [18] , [19] . The remaining seven genes were not induced by IFNγ/TLR and did not differ in WT and Irf8 −/− MФs ( Supplementary Fig. 2 ). These results indicate that many autophagy genes are induced by IFNγ/TLR stimulation in an IRF8-dependent manner. Rescue experiments in Fig. 1e showed that transfer of the Irf8 gene into Irf8 −/− MФs restored the expression of 10 autophagy genes on IFNγ/TLR stimulation. As expected, Irf8 transfer did not restore the expressions of these genes in unstimulated MФs. The transcriptionally defective mutant, Irf8K79E , in contrast, failed to rescue these autophagy genes. It is of note that Irf8 transfer did not rescue all 17 genes, which may be attributed to insufficient levels of IRF8 expression, insufficient post-translational changes in IRF8 proteins or other mechanisms. IRF8 binds to and stimulates autophagy genes in MФs Seven of the 17 autophagy genes upregulated by IRF8 carried IRF8-binding motifs within the 3.5-kb upstream promoter region ( Fig. 2a ) [19] , [33] . We performed qPCR-based chromatin immunoprecipitation (ChIP) analysis to test the binding of IRF8 to these genes in MФs. As shown in Fig. 2b , IRF8 bound to all seven genes in WT MФ, but not in Irf8 −/− MФs. IRF8 binding increased after IFNγ/TLR stimulation for most of the genes, consistent with enhanced mRNA expression after stimulation ( Fig. 1d ). Consistent with the expression data, Atg7 showed high IRF8 binding in UT WT MФs, and the expression fell slightly after stimulation. Figure 2c summarizes the data for mRNA expression, rescue by IRF8 and ChIP assay, illustrating that IRF8 stimulates transcription of many autophagy genes constitutively and after IFNγ/TLR stimulation. Figure 2: IRF8 binds to the promoters of autophagy genes. ( a ) Consensus IRF8-binding motifs are shown in bold on indicated autophagy gene promoters. ( b ) IRF8 binding to the above motifs was detected by ChIP for WT and Irf8 −/− MФs (UT or treated with IFNγ/TLR) normalized by normal IgG binding, and with β-globin as a negative control. Values represent the average of five independent experiments. * P ≤0.05 and ** P ≤0.01. (Student’s t -test). ( c ) Summary of qRT-PCR analysis rescue experiment and ChIP assays. Full size image Irf8 −/− MФs are defective in IFNγ/TLR-induced autophagy To test whether defective gene expression in Irf8 −/− MФs affects autophagic functions, we next examined the autophagosome formation in MФs expressing mCherry-enhanced green fluorescent protein (EGFP)-LC3B ( Fig. 3a ). This vector detects acid-sensitive (EGFP) and -resistant (mCherry) LC3, enabling us to assess the formation of autophagosomes and the subsequent fusion with lysosomes [34] . Before stimulation, GFP and mCherry signals were diffusely distributed over the cytoplasm both in WT and Irf8 −/− MФs. After IFNγ/TLR stimulation, GFP and mCherry signals relocalized to form prominent punctate structures representing autophagosomal vesicles in WT cells (see arrows in Fig. 3a ). In contrast, few fluorescent vesicles were seen in Irf8 −/− MФs. Quantification in Fig. 3a (lower panel) confirmed that the number of cells with fluorescent vesicles was much fewer in Irf8 −/− MФs. Deficiency in Irf8 −/− MФs to form LC3 vesicles was also evident with endogenous LC3 ( Supplementary Fig. 3a ). Electron microscopy analysis additionally showed a noticeable increase in autophagic vesicles in stimulated WT MФs, but not in Irf8 −/− MФs ( Fig. 3b , right panel) [35] . Immunoblot analysis was performed to assess phosphatidylethalamine conjugation of LC3 as detected by changes in LC3I and LC3II levels [36] . Cells were treated with bafilomycin A1 to block the fusion of autophagosomes to lysosomes [36] . Data in Fig. 3c (right panel) showed the amounts of LC3II increased in WT MФs after IFNγ/TLR stimulation. LC3II levels were significantly lower in Irf8 −/− MФs before stimulation and did not measurably increase after simulation, as confirmed by quantification ( Fig. 3c , right panel). Flow cytometric analysis to detect membrane-bound LC3 further validate these results, in that LC3 signals increased after stimulation in WT MФs. However, LC3 levels were lower in Irf8 −/− MФs before stimulation and remained low after stimulation ( Fig. 3d ) [37] . To ascertain whether IRF8 has a role in autophagosome–lysosome fusion and lysosomal clearance, immunoblot and flow cytometry assays were performed in the absence of bafilomycin A1 ( Supplementary Fig. 3b,c ) [36] . In WT MФs, the amounts of LC3 hardly increased after stimulation, suggesting lysosomal turnover of LC3. On the other hand, LC3 levels were again lower in Irf8 −/− MФs and the amounts were unchanged after stimulation. These data support the notion that IRF8 plays a role in autophagosome formation, and subsequent autophagolysosome formation and function in IFNγ/TLR-induced autophagy. Further supporting the role of IRF8 in autophagosome formation, the amounts of Atg5–Atg12 complex increased in WT MФs, but not in Irf8 −/− MФs on IFNγ/TLR stimulation ( Fig. 3e ). 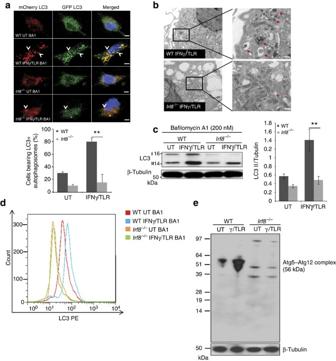Figure 3: Defective autophagosome formation inIrf8−/−MФs. (a) LC3 vesicles were visualized in WT andIrf8−/−MФs expressing mCherry-EGFP-LC3 vector, without (UT) or with IFNγ/TLR stimulation for 8 h. Bafilomycin A1 (BA1; 200 nM) was added for the final 2 h. Cells were counterstained for DNA (blue). Scale bar, 20 μm. Below: the number of cells with more than five mCherry-positive vesicles was counted by microscopic inspection of more than 200 cells. The values represent the percentage of cells with fluorescent vesicles. **P≤0.01 (Student’st-test). SeeSupplementary Fig. 3afor endogenous staining of LC3. (b) WT andIrf8−/−MФs treated with IFNγ overnight followed by TLR ligands for 8 h was inspected by transmission electron microscopy. The bracketed region in the left panel was enlarged in the right panel. Arrows indicate autophagic vacuoles. Scale bar, 0.5 μm. (c) Reduced LC3I to LC3II conversion inIrf8−/−MФs. WT andIrf8−/−MФs were treated with IFNγ/TLR as above with BA1 (200 nM) treatment for the final 2 h. Immunoblot analysis was performed with 10 μg of extracts with β-Tubulin as a control. Right panel: the amounts of LC3II in three independent samples were quantified using the ImageJ software. *P≤0.05 and **P≤0.01 (Student’st-test). SeeSupplementary Fig. 3bfor LC3 amount in the absence of BA1. (d) Membrane-bound LC3 in WT andIrf8−/−MΦs treated with IFNγ/TLR was detected by flow cytometry. BA1 (200 nM) was added for the final 2 h. The histogram is a representative of three independent experiments. SeeSupplementary Fig. 3cfor LC3 amount in the absence of BA1. (e) Immunoblot detection of the ATG5–ATG12 conjugate. WT andIrf8−/−MФs were treated as above and immunoblot detection of the ATG5–ATG12 conjugate proteins was performed. Ten micrograms of the extracts were tested with antibody against ATG5 or β-Tubulin. Figure 3: Defective autophagosome formation in Irf8 −/− MФs. ( a ) LC3 vesicles were visualized in WT and Irf8 −/− MФs expressing mCherry-EGFP-LC3 vector, without (UT) or with IFNγ/TLR stimulation for 8 h. Bafilomycin A1 (BA1; 200 nM) was added for the final 2 h. Cells were counterstained for DNA (blue). Scale bar, 20 μm. Below: the number of cells with more than five mCherry-positive vesicles was counted by microscopic inspection of more than 200 cells. The values represent the percentage of cells with fluorescent vesicles. ** P ≤0.01 (Student’s t -test). See Supplementary Fig. 3a for endogenous staining of LC3. ( b ) WT and Irf8 −/− MФs treated with IFNγ overnight followed by TLR ligands for 8 h was inspected by transmission electron microscopy. The bracketed region in the left panel was enlarged in the right panel. Arrows indicate autophagic vacuoles. Scale bar, 0.5 μm. ( c ) Reduced LC3I to LC3II conversion in Irf8 −/− MФs. WT and Irf8 −/− MФs were treated with IFNγ/TLR as above with BA1 (200 nM) treatment for the final 2 h. Immunoblot analysis was performed with 10 μg of extracts with β-Tubulin as a control. Right panel: the amounts of LC3II in three independent samples were quantified using the ImageJ software. * P ≤0.05 and ** P ≤0.01 (Student’s t -test). See Supplementary Fig. 3b for LC3 amount in the absence of BA1. ( d ) Membrane-bound LC3 in WT and Irf8 −/− MΦs treated with IFNγ/TLR was detected by flow cytometry. BA1 (200 nM) was added for the final 2 h. The histogram is a representative of three independent experiments. See Supplementary Fig. 3c for LC3 amount in the absence of BA1. ( e ) Immunoblot detection of the ATG5–ATG12 conjugate. WT and Irf8 −/− MФs were treated as above and immunoblot detection of the ATG5–ATG12 conjugate proteins was performed. Ten micrograms of the extracts were tested with antibody against ATG5 or β-Tubulin. Full size image We noted that although autophagy is linked to the downregulation of mammalian target of rapamycin (mTOR) kinase in a starvation model [1] , IFNγ/TLR stimulation did not downregulate phospho-mTOR expression, but it rather upregulated it in WT and Irf8 −/− MФs ( Supplementary Fig. 4 ), indicating that IFNγ/TLR-induced autophagy may not be directly controlled by mTOR activity, consistent with the recent report [5] . As autophagy proceeds further, autophagosomes fuse with lysosomes to become autolysosomes that carry LC3 and various lysosome-associated components [2] . LAMP2, a lysosomal membrane protein, is involved in the autophagosome–lysosome fusion [38] . Immunostaining and immunoblot data in Fig. 4a,b found that LAMP2 expression was lower in Irf8 −/− MФs than in the WT cells, consistent with reduced Lamp2 mRNA expression in Irf8 −/− cells ( Fig. 1d ). To test whether IRF8 affects autolysosome formation, we examined the co-localization of endogenous LC3 and lysosomes as detected by LysoTracker-red by immunostaining [36] . Immunostaining data in Fig. 4c showed that the majority of LC3 vesicles merged with LysoTracker-red staining in WT MФs on IFNγ/TLR stimulation (arrow heads). However, in Irf8 −/− MФs, LC3 and LysoTracker-red double positive vesicles were much fewer ( Fig. 4c ). These results indicate that through transcriptional control, IRF8 indirectly facilitates maturation of autophagosomes to autolysosomes in response to IFNγ/TLR stimulation. 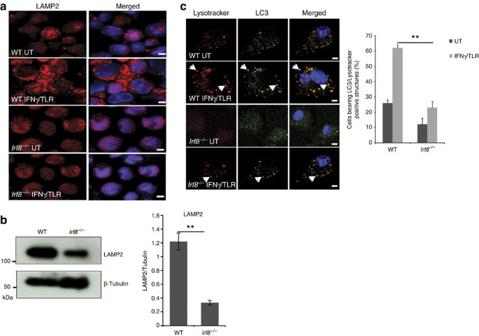Figure 4: Defective autophagosome maturation inIrf8−/−MФs. (a) Immunostaining of LAMP2 in WT andIrf8−/−MФs stimulated with IFNγ overnight and TLR ligands for 8 h. Cells were counterstained for DNA (blue). Scale bar, 20 μm. (b) Immunoblot detection of LAMP2 in WT andIrf8−/−MФs. Ten micrograms of extracts were tested with antibody against LAMP2 or β-Tubulin. Below: the amounts of LAMP2 in three independent experiments were quantified using the ImageJ software. **P≤0.01. (c) WT andIrf8−/−MФs were immunostained for LC3 antibody and LysoTracker-red to detect LC3-positive and lysosome-positive structures. Right: cells with double-positive vesicles were quantified as inFig. 3a. Data represent the average of three independent experiments.P≤0.01 (**). Scale bar, 20 μm. Figure 4: Defective autophagosome maturation in Irf8 −/− MФs. ( a ) Immunostaining of LAMP2 in WT and Irf8 −/− MФs stimulated with IFNγ overnight and TLR ligands for 8 h. Cells were counterstained for DNA (blue). Scale bar, 20 μm. ( b ) Immunoblot detection of LAMP2 in WT and Irf8 −/− MФs. Ten micrograms of extracts were tested with antibody against LAMP2 or β-Tubulin. Below: the amounts of LAMP2 in three independent experiments were quantified using the ImageJ software. ** P ≤0.01. ( c ) WT and Irf8 −/− MФs were immunostained for LC3 antibody and LysoTracker-red to detect LC3-positive and lysosome-positive structures. Right: cells with double-positive vesicles were quantified as in Fig. 3a . Data represent the average of three independent experiments. P ≤0.01 (**). Scale bar, 20 μm. Full size image Irf8 −/− MФs accumulate SQSTM1/ubiquitinated proteins Misfolded self-proteins and invading pathogens are often conjugated to ubiquitin and escorted to autophagosomes to be degraded in lysosomes. This process is partly mediated by the ubiquitin adaptor SQSTM1 (p62) [13] , [14] . Some autophagy-deficient cells form aggregates, called aggresomes or inclusion bodies that contain SQSTM1 and ubiquitin [14] . In light of defective autophagy, it was possible that Irf8 −/− MФs abnormally accumulate SQSTM1 and ubiquitin-containing proteins. Immunostaining of ubiquitin and SQSTM1 showed extensive deposition of SQSTM1 that co-localized with ubiquitin-positive proteins in Irf8 −/− MФs after IFNγ/TLR stimulation, in contrast to WT MФs that showed little deposition of these proteins ( Fig. 5a , left panel). Quantification of SQSTM1 and ubiquitin-positive cells confirmed the immunostaining results ( Fig. 5a , right panel). Immunoblot analysis further confirmed that SQSTM1 accumulates in greater amounts in Irf8 −/− than WT MФs with and without bafilomycin A1 treatment ( Fig. 5b upper panel and Supplementary Fig. 3b ). In addition, the amounts of ubiquitin-positive proteins increased markedly after stimulation and to a greater extent in Irf8 −/− MФs than WT cells ( Fig. 5b , left and right panels). In agreement with the increased ubiquitin-positive proteins, we previously noted that IFNγ/TLR stimulation increases ubiquitin-conjugated proteins in MФs [39] . Next, we tested whether the larger increase in SQSTM1 protein expression in Irf8 −/− cells was due to higher Sqstm1 transcription in Irf8 −/− MФs. Relevant to this question, we previously showed that Sqstm1 mRNA expression increases after IFNγ/TLR stimulation in WT MФs [40] . qRT–PCR data showed that the levels of Sqstm1 mRNA were comparable in WT and Irf8 −/− MФs, indicating that SQSTM1 proteins aberrantly accumulate in Irf8 −/− cells after stimulation, due to deficiency in autophagic degradation ( Supplementary Fig. 5 ). To ascertain the role of autophagic degradation in the elimination of ubiquitin-conjugated proteins, in addition to proteasome mediated degradation, immunoblot analysis was performed for cells treated with a proteasome inhibitor, MG132. As seen in Fig. 5c left and right panels, Irf8 −/− MФs accumulated greater amounts of ubiquitin-bound proteins than WT MФs in the presence of MG132, suggesting that autophagy partly accounted for excess accumulation of SQSTM1 and ubiquitin-bound proteins in Irf8 −/− MФs. Further supporting the accumulation of unprocessed proteins in Irf8 −/− MФs, MitoTracker-positive materials that co-localized with monodansylcadaverine staining were more abundant in Irf8 −/− MФs than WT cells ( Supplementary Fig. 6 ) [36] . 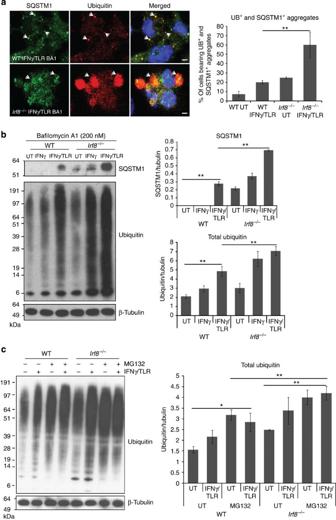Figure 5: SQSTM1 and ubiquitin-conjugated proteins form aggregates inIrf8−/−MΦs. (a) SQSTM1- and ubiquitin-positive proteins (arrow heads) in WT andIrf8−/−MФs stimulated with IFNγ overnight and TLR ligands for 8 h were visualized by immunostaining. Bafilomycin A1 (200 nM) was added for the final 2 h. Cells were counterstained for DNA (blue). Right panel: the percentage of cells with SQSTM1- and ubiquitin-positive aggregates. Data represent the average of three independent experiments ±s.d. with **P≤0.01 (Student’st-test). (b) Immunoblot detection of SQSTM1- and ubiquitin-positive proteins in WT andIrf8−/−MФs stimulated with IFNγ or IFNγ/TLR for 8 h. Bafilomycin A1 (200 nM) was added for the final 2 h. Right panel: relative amounts of ubiquitin-bound proteins. Data represent the average of three independent experiments ±s.d. with **P≤0.01 (Student’st-test). SeeSupplementary Fig. 3bfor immunoblot detection of SQSTM1 in the absence of bafilomycin A1. (c) Immunoblot detection of ubiquitin-bound proteins in the presence of MG132. WT andIrf8−/−MФs were stimulated with IFNγ/TLR in the presence of 10 μM of MG132. Right panel: relative amounts of ubiquitin-bound proteins. Data represent the average of three independent experiments ±s.d. with *P≤0.05 and **P≤0.01 (Student’st-test). Figure 5: SQSTM1 and ubiquitin-conjugated proteins form aggregates in Irf8 −/− MΦs. ( a ) SQSTM1- and ubiquitin-positive proteins (arrow heads) in WT and Irf8 −/− MФs stimulated with IFNγ overnight and TLR ligands for 8 h were visualized by immunostaining. Bafilomycin A1 (200 nM) was added for the final 2 h. Cells were counterstained for DNA (blue). Right panel: the percentage of cells with SQSTM1- and ubiquitin-positive aggregates. Data represent the average of three independent experiments ±s.d. with ** P ≤0.01 (Student’s t -test). ( b ) Immunoblot detection of SQSTM1- and ubiquitin-positive proteins in WT and Irf8 −/− MФs stimulated with IFNγ or IFNγ/TLR for 8 h. Bafilomycin A1 (200 nM) was added for the final 2 h. Right panel: relative amounts of ubiquitin-bound proteins. Data represent the average of three independent experiments ±s.d. with ** P ≤0.01 (Student’s t -test). See Supplementary Fig. 3b for immunoblot detection of SQSTM1 in the absence of bafilomycin A1. ( c ) Immunoblot detection of ubiquitin-bound proteins in the presence of MG132. WT and Irf8 −/− MФs were stimulated with IFNγ/TLR in the presence of 10 μM of MG132. Right panel: relative amounts of ubiquitin-bound proteins. Data represent the average of three independent experiments ±s.d. with * P ≤0.05 and ** P ≤0.01 (Student’s t -test). Full size image IRF8 is required for autophagic clearance of Listeria Autophagy is a major mechanism by which MФs eliminate intracellular bacteria, such as M. tuberculosis , Salmonella and Listeria [6] , [10] , [41] . Previous studies showed that IRF8 is essential for controlling infection of the above bacteria [22] , [23] , [24] , [25] , [26] . However, it has not been clear whether IRF8 employs autophagy to confer protection. We first examined whether Listeria infection activates autophagy genes in MФs: Listeria monocytogenes is a food-borne pathogen that causes listeriosis and is widely studied in mouse models [42] . qRT–PCR data in Fig. 6a showed that the expression of Listeria transcripts rose sharply in Irf8 −/− MФs during 48 h of infection, while remained very low in WT MФs, including ActA shown to bypass host cell autophagy [41] . On the other hand, Listeria infection markedly increased expression of many autophagy genes in WT MФs, in some cases by nearly 100-folds ( Fig. 6b ). Among induced genes was Nod1 , important for autophagy-mediated control of Listeria [43] . Interestingly, on Listeria infection, Irf8 expression was also dramatically increased. In contrast, none of these autophagy genes were induced in Irf8 −/− MФs at comparable levels ( Fig. 6b ). Accordingly, while WT MФs restricted bacterial growth to a minimum, Irf8 −/− MФs relented to the logarithmic growth of Listeria , as verified by bacterial accumulation in the cytoplasm ( Fig. 6c ). Further supporting IRF8-dependent autophagic activation, LC3II levels increased during Listeria infection in WT MФs but not in Irf8 −/− MФs, as observed in the presence of bafilomycin A1 ( Fig. 6d ). In contrast, LC3II amounts remained much lower in Irf8 −/− MФs during infection. In the absence of bafilomycin A1, LC3II amounts increased at 24 h, then gradually decreased afterwards up to 48 h ( Supplementary Fig. 7a ) in WT MФs. In Irf8 −/− MФs, LC3II amounts also increased at 24 h, but remained high throughout 48 h of infection, suggesting inefficient LC3 turnover in lysosomes [36] , [44] . In agreement, SQSTM1 and SQSTM1-positive proteins accumulated in Irf8 −/− MФs in greater amounts than WT cells with and without bafilomycin A1 ( Fig. 6d , Supplementary Fig. 7a ). Together these results reinforce the view that during Listeria infection, IRF8 plays a major role in promoting both autophagosome formation and the subsequent autolysosomal functions. Importantly, immunostaining analysis in Fig. 6e revealed that Listeria antigens co-localized with LC3 and formed autophagosomal vesicles in WT cells, indicative of autophagic capturing of bacterial antigens. However, the Listeria antigens were more abundant in Irf8 −/− MФs than in WT cells and the co-localization with LC3 was hardly observed ( Fig. 6e ). We also found that blocking of autophagosome–lysosome fusion by bafilomycin A1 led to logarithmic growth of Listeria in WT MФs, comparable to that in Irf8 −/− MФs, supporting autophagic control of Listeria infection ( Fig. 6c ). To ascertain whether autophagic control of Listeria relies on de novo transcription of autophagy genes, infected WT and Irf8 −/− MФs were briefly treated with Actinomycin D (Act D) and tested for bacterial growth. As shown in Fig. 6f , bacterial counts sharply increased after 2 h of Act D treatment both in WT and Irf8 −/− MФs. Act D also inhibited autophagosome formation and expression of autophagy genes on IFNγ/TLR stimulation ( Supplementary Fig. 8 ). These results are analogous to the previous report where muscle cell autophagy depends on FOXO3-mediated transcription of autophagy genes [17] . 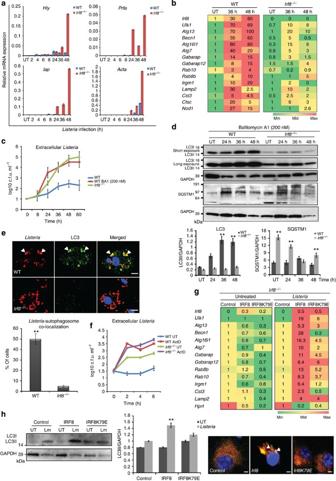Figure 6: IRF8 is required for the autophagic clearance ofListeria. (a) WT andIrf8−/−MФs (106) were infected withListeria(5 × 107) and bacterial transcripts were detected by qRT–PCR, normalized byGapdh. Data represent the average of three independent experiments.P≤0.05 (Student’st-test). (b) Autophagy gene expression in indicated MФs was detected as above and normalized to those in uninfected WT MΦs. Data represent the average of three independent experiments.P≤0.05 (Student’st-test). (c) Bacterial yields tested by the colony-forming unit (c.f.u.) assay. Some WT MФs were treated with bafilomycin A1 (200 nM). Values represent the average of three determinations ±s.d. (d) Immunoblot analysis of LC3 and SQSTM1 inListeria-infected WT andIrf8−/−MФs in the presence of bafilomycin A1 (200 nM). Below: amounts of LC3 and SQSTM1 from three independent samples were quantified by ImageJ software. **P≤0.01 (Student’st-test). SeeSupplementary Fig. 7afor LC3 and SQSTM1 amounts in the absence of bafilomycin A1. (e) Distribution ofListeriaantigens and LC3 after 36 h ofListeriainfection in immunostaining. Arrow heads: LC3-associatedListeria. Scale bar, 20 μm. Below: the percentage of cells showing the co-localization of LC3 andListeriaantigens. Values represent the average of three independent experiments ±s.d. with **P≤0.01 (Student’st-test). (f) Bacterial yields in MФs infected withListeriafor 24 h and treated with Act D (2 μg ml−1). Data represent the average of three determinations ±s.d. SeeSupplementary Fig. 8for details of Act D effects. (g)Irf8−/−MФs transduced withIrf8vector were infected withListeriafor 36 h and autophagy gene expression was detected as above. The numbers represent transcript levels normalized by those with empty vector.Irf8transcripts were normalized bygapdh. Values are the average of three experiments.P≤0.05 (Student’st-test).Hprt: a negative control. (h) Left and middle:Irf8−/−MФs transduced as above were tested for LC3II using GAPDH as a control. The amounts of LC3II in two independent experiments were quantified using ImageJ software. **P≤0.01 (Student’st-test). Right:Irf8−/−MФs expressing mCherry-EGFP-LC3 were transduced as above and infected withListeriafor 36 h and fluorescent LC3 signals was visualized by confocal microscopy. SeeSupplementary Fig. 7bfor microscopy image with controls. Figure 6: IRF8 is required for the autophagic clearance of Listeria . ( a ) WT and Irf8 −/− MФs (10 6 ) were infected with Listeria (5 × 10 7 ) and bacterial transcripts were detected by qRT–PCR, normalized by Gapdh . Data represent the average of three independent experiments. P ≤0.05 (Student’s t -test). ( b ) Autophagy gene expression in indicated MФs was detected as above and normalized to those in uninfected WT MΦs. Data represent the average of three independent experiments. P ≤0.05 (Student’s t -test). ( c ) Bacterial yields tested by the colony-forming unit (c.f.u.) assay. Some WT MФs were treated with bafilomycin A1 (200 nM). Values represent the average of three determinations ±s.d. ( d ) Immunoblot analysis of LC3 and SQSTM1 in Listeria -infected WT and Irf8 −/− MФs in the presence of bafilomycin A1 (200 nM). Below: amounts of LC3 and SQSTM1 from three independent samples were quantified by ImageJ software. ** P ≤0.01 (Student’s t -test). See Supplementary Fig. 7a for LC3 and SQSTM1 amounts in the absence of bafilomycin A1. ( e ) Distribution of Listeria antigens and LC3 after 36 h of Listeria infection in immunostaining. Arrow heads: LC3-associated Listeria . Scale bar, 20 μm. Below: the percentage of cells showing the co-localization of LC3 and Listeria antigens. Values represent the average of three independent experiments ±s.d. with ** P ≤0.01 (Student’s t -test). ( f ) Bacterial yields in MФs infected with Listeria for 24 h and treated with Act D (2 μg ml −1 ). Data represent the average of three determinations ±s.d. See Supplementary Fig. 8 for details of Act D effects. ( g ) Irf8 −/− MФs transduced with Irf8 vector were infected with Listeria for 36 h and autophagy gene expression was detected as above. The numbers represent transcript levels normalized by those with empty vector. Irf8 transcripts were normalized by gapdh . Values are the average of three experiments. P ≤0.05 (Student’s t -test). Hprt : a negative control. ( h ) Left and middle: Irf8 −/− MФs transduced as above were tested for LC3II using GAPDH as a control. The amounts of LC3II in two independent experiments were quantified using ImageJ software. ** P ≤0.01 (Student’s t -test). Right: Irf8 −/− MФs expressing mCherry-EGFP-LC3 were transduced as above and infected with Listeria for 36 h and fluorescent LC3 signals was visualized by confocal microscopy. See Supplementary Fig. 7b for microscopy image with controls. Full size image Rescue experiments in Fig. 6g showed that transfer of the WT Irf8 gene into Irf8 −/− MФs restored expression of most of the autophagy genes induced by Listeria shown in Fig. 6b . In contrast, none of these genes were rescued by the mutant Irf8K79E ( Fig. 6g ). Furthermore, transfer of WT Irf8 , but not the mutant, restored the ability to increase LC3II protein expression after Listeria infection ( Fig. 6h , left and middle panels). Consequently, Irf8 gene transfer led to a marked increase in LC3-positive vesicles ( Fig. 6h , right panel and Supplementary Fig. 7b ). These data provide strong evidence that IRF8-dependent transcription plays a major role in autophagic control of Listeria infection in MФs. IRF8 regulates starvation and M-CSF-induced autophagy Starvation is one of the best-studied autophagy models [1] . Because starvation is seemingly unrelated to innate immunity, and have not been studied extensively in MФs, we asked whether starvation induces autophagy in MФs and if so, whether IRF8 plays a role. We found that many autophagy genes were induced in WT MФs on starvation, although the pattern of induction differed from that seen by IFNγ/TLR or Listeria infection ( Fig. 7a ). Notably, the genes active in early stages of autophagy were induced after starvation, whereas those involved in later stages were not. Moreover, Irf8 itself was also induced after starvation in WT cells, although modestly. In contrast, these genes were not induced in Irf8 −/− MФs at comparable levels. Basal expression of many autophagy genes was also lower in Irf8 −/− MФs than WT cells. Interestingly, Tfeb , a master regulator of starvation-induced autophagy, involved in lysosomal biogenesis, was induced in MФs in an IRF8-dependent manner [16] . On the other hand, Foxo3 , the transcription factor that regulates autophagy in atrophying muscle cells was expressed at similar levels in WT and Irf8 −/− MФs, and was not induced by any of the stimuli tested in this study ( Supplementary Fig. 9 ) [17] . 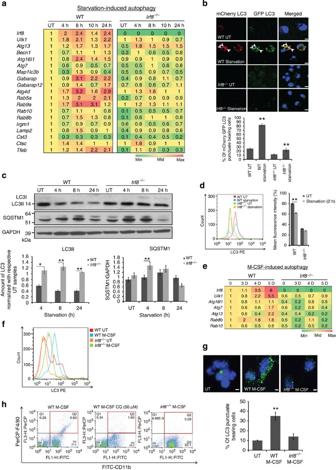Figure 7: IRF8 stimulates starvation and M-CSF-induced autophagy. (a) Autophagy gene expression in WT andIrf8−/−MФs after starvation was detected by qRT–PCR and normalized by transcript values in UT WT cells. The number represents the average of three independent experiments.P≤0.05 (Student’st-test). (b) WT andIrf8−/−MФs expressing mCherry-EGFP-LC3 after starvation for 6 h and LC3 fluorescence signals (arrow heads) were visualized. Below: the percentage of cells with double-positive LC3 signals. Data represent the average of three independent experiments. **P≤0.01 (Student’st-test). Scale bar, 20 μm. SeeSupplementary Fig. 10dfor LC3 fluorescence signals in the presence of bafilomycin A1. (c) Immunoblot detection of LC3II and SQSTM1 in starved WT andIrf8−/−MФs. Below: the amounts of total LC3 and SQSTM1 in three independent samples quantified by ImageJ software. *P≤0.05 and **P≤0.01 (Student’st-test). SeeSupplementary Fig. 10cfor LC3 and SQSTM1 amounts in the presence of bafilomycin A1. (d) Left panel: membrane-bound LC3 in WT andIrf8−/−MФs after 2 h starvation was detected by flow cytometry. The histogram is a typical example of three independent experiments. Right panel: mean fluorescence intensity of membrane-bound LC3. Values represent the mean of three independent experiments. **P≤0.01 (Student’st-test). SeeSupplementary Fig. 10efor fluorescence-activated cell sorting detection in the presence of bafilomycin A1. (e) Autophagy gene expression in WT andIrf8−/−BM cells cultured in M-CSF was detected by qRT–PCR, and transcripts were normalized by values in WT cells on day 0. The number represents the average of three independent experiments.P≤0.05 (Student’st-test). (f) Membrane-bound LC3 in WT andIrf8−/−MΦs cultured in M-CSF for 4 days was detected by flow cytometry. The histogram is a typical example of three independent experiments. Similar results were observed with MΦs on days 3 and 5 (SeeSupplementary Fig. 11a). (g) LC3 vesicles in WT andIrf8−/−MΦs cultured in M-CSF for 3 days was detected by immunostaining. Below: the percentage of cells bearing LC3 vesicles. **P≤0.01 (Student’st-test). Scale bar, 20 μm. (h) Expression of F4/80 and CD11b was detected in WT andIrf8−/−MΦs cultured in M-CSF for 3 days by flow cytometry. Chloroquine (50 μM) was added in the middle panel for the final 18 h. Similar results were observed in three independent experiments. Figure 7: IRF8 stimulates starvation and M-CSF-induced autophagy. ( a ) Autophagy gene expression in WT and Irf8 −/− MФs after starvation was detected by qRT–PCR and normalized by transcript values in UT WT cells. The number represents the average of three independent experiments. P ≤0.05 (Student’s t -test). ( b ) WT and Irf8 −/− MФs expressing mCherry-EGFP-LC3 after starvation for 6 h and LC3 fluorescence signals (arrow heads) were visualized. Below: the percentage of cells with double-positive LC3 signals. Data represent the average of three independent experiments. ** P ≤0.01 (Student’s t -test). Scale bar, 20 μm. See Supplementary Fig. 10d for LC3 fluorescence signals in the presence of bafilomycin A1. ( c ) Immunoblot detection of LC3II and SQSTM1 in starved WT and Irf8 −/− MФs. Below: the amounts of total LC3 and SQSTM1 in three independent samples quantified by ImageJ software. * P ≤0.05 and ** P ≤0.01 (Student’s t -test). See Supplementary Fig. 10c for LC3 and SQSTM1 amounts in the presence of bafilomycin A1. ( d ) Left panel: membrane-bound LC3 in WT and Irf8 −/− MФs after 2 h starvation was detected by flow cytometry. The histogram is a typical example of three independent experiments. Right panel: mean fluorescence intensity of membrane-bound LC3. Values represent the mean of three independent experiments. ** P ≤0.01 (Student’s t -test). See Supplementary Fig. 10e for fluorescence-activated cell sorting detection in the presence of bafilomycin A1. ( e ) Autophagy gene expression in WT and Irf8 −/− BM cells cultured in M-CSF was detected by qRT–PCR, and transcripts were normalized by values in WT cells on day 0. The number represents the average of three independent experiments. P ≤0.05 (Student’s t -test). ( f ) Membrane-bound LC3 in WT and Irf8 −/− MΦs cultured in M-CSF for 4 days was detected by flow cytometry. The histogram is a typical example of three independent experiments. Similar results were observed with MΦs on days 3 and 5 (See Supplementary Fig. 11a ). ( g ) LC3 vesicles in WT and Irf8 −/− MΦs cultured in M-CSF for 3 days was detected by immunostaining. Below: the percentage of cells bearing LC3 vesicles. ** P ≤0.01 (Student’s t -test). Scale bar, 20 μm. ( h ) Expression of F4/80 and CD11b was detected in WT and Irf8 −/− MΦs cultured in M-CSF for 3 days by flow cytometry. Chloroquine (50 μM) was added in the middle panel for the final 18 h. Similar results were observed in three independent experiments. Full size image Rescue experiments in Supplementary Fig. 10a showed that transfer of WT Irf8, but not Irf8K79E mutant into Irf8 −/− MФs restored the expression of five autophagy genes during starvation condition. Thus, starvation activates transcription of multiple autophagy genes in MФs in an IRF8-dependent manner. We next examined mCherry-EGFP-LC3 fluorescent signals after starvation and found many fluorescence-positive vesicles in WT MФs, while only diffuse signals in Irf8 −/− MФs, indicating that starvation induces autophagosome formation in WT MФs, but this process is severely impaired in Irf8 −/− MФs ( Fig. 7b , see quantification below). LC3 flux analysis in Fig. 7c showed that the amount of LC3II fell 8 and 24 h after starvation in WT MФs. Whereas, the amounts of LC3 remained similar in Irf8 −/− MФs under these conditions, suggesting that LC3 was autophagically processed in WT MФs as reported for other cells, and this process was defective in Irf8 −/− MФs [44] ( Fig. 7c top and bottom). Consistent with the immunoblot data, flow cytometry analysis in Fig. 7d found that amounts of membrane-bound LC3 were reduced after starvation in WT MФs, but not in Irf8 −/− MФs. Cell viability assay confirmed that the reduced LC3 amounts in WT MФs during starvation were not due to toxicity of nutrient deprivation ( Supplementary Fig. 10b ). Above assays were performed in the absence of bafilomycin A1. To assess the role of IRF8 in autophagosome formation, we performed similar assays in the presence of bafilomycin A1. In immunoblot assays, amounts of LC3II appeared similar in WT MФs and Irf8 −/− MФs after starvation ( Supplementary Fig. 10c ). These data support lysosomal processing of LC3 in WT MФs as suggested above. Nonetheless, the results differed from those seen by all other stresses tested, including M-CSF (below), in which LC3II levels were lower in Irf8 −/− MФs than WT MФs in the presence of bafilomycin A1. This difference may be due to differential influence of IRF8 on LC3II protein levels under different stresses. Importantly, however, EGFP-positive punctae as well as membrane-bound LC3 were markedly lower in Irf8 −/− MФs relative to WT MФs in the presence of bafilomycin A1 (see microscopy and flow cytometry data in Supplementary Fig. 10d,e ). Overall, these results point to a deficiency in forming intact autophagosomes in Irf8 −/− MФs in addition to defects in the subsequent steps such as lysosomal fusion and protein processing. Further, we found that the amounts of SQSTM1 were higher in Irf8 −/− MФs than WT MФs during 8 h of starvation both with or without bafilomycin A1 ( Fig. 7c and Supplementary Fig. 10c ). We also found that starvation downregulated phospho-mTOR in WT and Irf8 −/− MФs ( Supplementary Fig. 10f ), as shown in other cell types [1] ( Supplementary Fig. 4 ). Thus, Irf8 −/− MФs, although capable of downregulating mTOR on starvation, are nevertheless defective in starvation-induced autophagy. Recent reports document that autophagy promotes M-CSF-mediated monocyte to MФ differentiation in vitro [11] , [12] . In view of the fact that IRF8 drives MФ differentiation, it was of interest to test whether IRF8 affects M-CSF-mediated autophagy during MФ maturation [19] , [21] . qRT–PCR analysis in Fig. 7e showed that expression of various autophagy genes increased during 5 days of WT BM cell cultures with M-CSF. In contrast, none of these genes were induced in Irf8 −/− cells. Irf8 was strongly induced in WT cells cultured in M-CSF [33] . Flow cytometric analysis showed that membrane-bound LC3 signals increased in WT cell cultures, but only modestly in Irf8 −/− cell cultures ( Fig. 7f and Supplementary Fig. 11a ). LC3 signals in UT cells were also lower in Irf8 −/− cells than WT cells. Furthermore, immunostaining analysis in Fig. 7g showed that the number of cells with LC3 vesicles was noticeably higher in WT cells than Irf8 −/− cells. In accordance, immunoblot analysis showed that the levels of LC3II increased in WT cells during M-CSF, but in Irf8 −/− cells LC3 levels only meagerly increased with or without bafilomycin A1, indicating defective autophagosome formation and fusion with lysosomes ( Supplementary Fig. 11b ). The amounts of SQSTM1 were higher in M-CSF treated Irf8 −/− cells as compared with WT cells also with and without bafilomycin A1, suggesting greater accumulation of SQSTM1 in Irf8 −/− cells than WT cells ( Supplementary Fig. 11b ). As expected, WT cell cultures generated many more cells expressing authentic MФ markers, F4/80 and CD11b, compared with Irf8 −/− cell cultures ( Fig. 7h ). Treatment with Chloroquine to inhibit autolysosome function led to a marked reduction in F4/80 and CD11b-positive cells ( Fig. 7h ). These results support a role for autophagy in M-CSF-mediated MФ differentiation in which IRF8 plays an important part. In this study, we show that IRF8 stimulates a series of autophagy genes on various stresses known to activate autophagy in MФs, including IFNγ/TLR, Listeria infection, starvation and M-CSF stimulation. Consequently, IRF8 was found to play a critical role in autophagic progression, from autophagosome formation to autolysosomes and degradation of cellular components. Moreover, on Listeria infection, IRF8 critically contributed to the elimination of the intracellular bacteria. It is clear that IRF8, although not an autophagy effector by itself, is indispensable for the execution of autophagy in MФs. In most cases, autophagy genes regulated by IRF8 ranged widely, covering essentially the entire autophagic pathways, from the initial autophagosome activation to the final lysosomal degradation of captured targets, indicating that IRF8 influences autophagic events from the beginning to the end. Because many of autophagy genes were transcriptionally activated on stress in MФs, efficient autophagic execution in these cells must require transcriptional input. Our data show that IRF8 activates transcription of autophagy genes directly or in cooperation with other factors, since (a) IRF8 bound to the promoter of multiple autophagy genes and (b) expression of these and additional autophagy genes was rescued by Irf8 gene transfer in Irf8 −/− MФs. Consequently, Irf8 −/− MФs were impaired in many autophagic functions, ranging from defective autophagosome formation to autophagic degradation of cellular components, including ubiquitin-bound proteins such as SQSTM1. Most importantly, Irf8 −/− MФs were unable to control the growth of Listeria . On the basis of the central role that IRF8 plays in all autophagy settings we tested, IRF8 may be regarded as one of the master regulators of MΦ autophagy. In many cases, autophagy is likely to be initiated by the preexisting cytoplasmic autophagy effectors. Nevertheless, some autophagy components are presumably turned over to be replaced by newly synthesized components. There are a few examples where proteins required for autophagy are synthesized during autophagic events by distinct transcription factors [16] , [17] . For example, muscle atrophy-associated autophagy requires FOXO3, a transcription factor of the forkhead family [17] . FOXO3 is activated by starvation and it then induces a number of autophagy genes to stimulate lysosomal proteolysis, which leads to the degradation of cellular components and muscle cell atrophy. Second, TFEB, a transcription factor of the bHLH family, regulates genes important for biogenesis and functions of lysosomes. Through this action, TFEB coordinates autophagy-mediated lipid metabolism [16] . In these cases, FOXO3 and TFEB provide a mechanism to coordinate autophagic processes. The function of IRF8 in MФ autophagy found in this study is comparable to those of FOXO3 and TFEB, although these factors act on different aspects of autophagy in different cell types. The above reports, combined with our results, lead us to a line of thinking that activities of individual autophagy genes are organized as a network by a central regulator that integrates separate autophagic events to achieve orderly elimination of target factors. FOXO3 and TFEB may thus represent the founding members of autophagy master regulators. It is not surprising that autophagy master regulators so far identified are transcription factors, given that they regulate multiple genes in a signal-dependent manner. 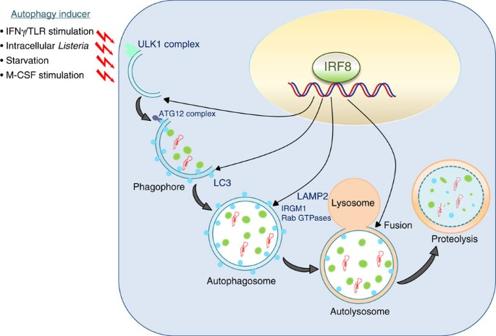Figure 8: A model for IRF8-dependent autophagy in MΦs. On various stresses (IFNγ/TLR stimulation,Listeriainfection, starvation and M-CSF stimulation), IRF8 is activated and promotes the expression of a series of autophagy genes. These genes encode factors active at various stages of autophagy, largely covering the whole autophagic cascade.Irf8−/−MΦs are defective in autophagic activation and fail to degrade target ubiquitin-conjugated factors, organelle and intracellular pathogens. Together, IRF8 acts as an autophagy master regulator in MΦs to coordinate stress responses critical for innate immunity. Figure 8: A model for IRF8-dependent autophagy in MΦs. On various stresses (IFNγ/TLR stimulation, Listeria infection, starvation and M-CSF stimulation), IRF8 is activated and promotes the expression of a series of autophagy genes. These genes encode factors active at various stages of autophagy, largely covering the whole autophagic cascade. Irf8 −/− MΦs are defective in autophagic activation and fail to degrade target ubiquitin-conjugated factors, organelle and intracellular pathogens. Together, IRF8 acts as an autophagy master regulator in MΦs to coordinate stress responses critical for innate immunity. Full size image While IRF8 was important for the execution of autophagy after varying stresses, we noted that the patterns of autophagy gene induction varied under different stress conditions. For example, Atg7 , downregulated by IFNγ/TLR and starvation was, however, upregulated by Listeria infection. In addition, the range of autophagy genes rescued by Irf8 gene transfer varied among different stresses. Moreover, IRF8 influenced LC3II levels in starvation differently from other stresses. Autophagic competence is a vital requirement for the function and survival of MФs and DCs, since these cells, acting as sentinels, must detect and eliminate invading pathogens rapidly. MФs and DCs thus produce a large amount of reactive oxygen species and nitric oxide as part of the antimicrobial defense. These compounds, however, as free radicals, likely damage the integrity of cellular components, which need to be processed in a timely manner. IRF8 was induced by classic stresses, IFNγ/TLR, starvation and Listeria infection. Although not regarded as a classic stress factor, M-CSF too may involve some types of stress, given that it activates the stress kinase JNK [12] . Thus, one could envisage that IRF8 may be adopted by MФs and DCs to meet heightened requirement for responding to stresses by augmenting autophagic functions. It was striking that Listeria infection caused a dramatic and prolonged expression of many autophagy genes along with that of Irf8 itself. The high, sustained expression of autophagy genes indicate that many autophagy factors were newly synthesized and replenished in MФs during infection in an IRF8-dependent manner to support autophagic control of bacterial growth. Our observation that a brief Act D treatment gave way to rapid bacterial growth in WT MФs may further support the view that continuous autophagy gene transcription is required for sustained resistance to Listeria infection. Furthermore, our results that LC3 co-localized with Listeria antigens are consistent with the report that autophagy plays a critical role in combating Listeria infection by linking ubiquitin pathways [45] . Moreover, our observations that Irf8 gene transfer led to a partial rescue of autophagosome formation provide compelling evidence that IRF8-dependent transcription critically contributes to the control of Listeria infection in MΦs. It is noteworthy that IRF8 has been known to play a crucial role in combating Listeria infection since 1997 (ref. 23 ). Our results are consistent with this early study and provide deeper insight into the mechanism by which IRF8 confers resistance to the bacteria. In a similar context, it has been shown that IRF8 is essential for controlling infection by other bacteria, including M. tuberculosis: mutations in Irf8 are associated with increased susceptibility to Mycobacteria infection in mice and humans [24] , [25] , [26] . However, underlying molecular mechanisms have not been fully clarified. In light of recent reports that autophagic clearance is critically required for controlling Mycobacteria infection, it seems likely that autophagy is an important means by which IRF8 exerts antimycobacterium activity [6] , [7] . IRF8 may also augment other aspects of innate immunity through autophagy, such as major histocompatibility complex II-mediated antigen presentation to TLR-dependent type I IFN induction [4] , [9] . In conclusion, IRF8 activates autophagic cascades in MФs at the level of transcription, and orchestrates capturing and elimination of endogenous targets and infectious pathogens. Mice and cells WT and Irf8 −/− mice on C57BL/6 background [18] were maintained in the NICHD animal facility. All animal work conformed to the NICHD animal care and use committee guidelines. BM mononuclear cells isolated from age-matched mice (female, 6–10 weeks old) were cultured as described previously [20] . In brief, BM mononuclear cells were cultured in complete RPMI medium (RPMI, 10% fetal bovine serum, 1 mM sodium pyruvate, 0.1 mM NEAA, 0.05 mM β-mercaptoethanol, 2 mM L -glutamine, 100 U ml −1 streptomycin/penicillin) in the presence of Flt3L (100 ng ml −1 ) or M-CSF (20 ng ml −1 ) for 5 to 6 days to generate DCs and MФs, respectively. DCs were stimulated with 100 ng ml −1 of LPS (Sigma) and 1 μg ml −1 of CpG 1826 (Lofstrand Labs) for 4–6 h for microarray analysis. MΦs were treated with IFNγ (100 U ml −1 ) overnight followed by stimulation with LPS (100 ng ml −1 ) and CpG 1826 (1 μg ml −1 ) for indicated periods. For starvation, MФs were washed with PBS and incubated in Earle’s balanced salt solution at 37 °C for indicated times. In some cases, MФs were treated with Act D (Sigma, cat. no. A1410) at 2 μg ml −1 for indicated times. For bacterial infection, MΦs were stimulated with IFNγ (100 U ml −1 ) in antibiotics free media for 20 h followed by infection with Listeria monocytogenes 10403S at a bacteria to cell ratio of 50:1 and maintained in complete media for indicated times [46] . Bacterial yields were measured by colony-forming unit assay after plating serially diluted culture supernatants of infected cells on BHI agar (Sigma, cat. no. 70138). For M-CSF treatment, BM-derived mononuclear cells were incubated in media containing MФ-colony-stimulating factor (M-CSF (Peprotech), 20 ng ml −1 ) at 37 °C for indicated days. Microarray analysis Total RNA from unstimulated and TLR-stimulated DCs was processed through RNeasy column (Qiagen) to remove possible DNA contaminants. Two independent RNA samples prepared from UT and TLR-stimulated DCs of WT and Irf8 −/− mice were subjected to microarray analysis using the Affymetrix Genechip Mouse 430 A 2.0 through Cogenics Inc. In brief, 1 μg of total RNA was converted to double-stranded complementary DNA with the Bioarray Single-Round RNA Amplification and Labeling Kit (Enzo Life Sciences) and multiple copies of biotinylated cRNA were synthesized by in vitro transcription with the Bioarray HighYield RNA Transcript Labeling Kit (Enzo Life Sciences), and assessed for quality by an Agilent Bioanalyzer. Six and a half μg of biotinylated cRNA spiked with bioB, bioC, bioD was hybridized to the array for 16 h at 45 °C. Arrays were washed, stained in an Affymetrix GeneChip Fluidics Station and scanned with an Affymetrix GeneChip Scanner 3000. Quality checks and data analyses were carried out using Affymetrix GeneChip Operating Software (GCOS) and Expression Console. All arrays have passed Cogenics’ internal QC metrics. Values with P ≤0.05 and two-fold cutoff were considered significant. Analysis of variance (including t -tests), was used to identify differentially expressed genes [28] . Raw data files have been deposited in the NCBI Gene Expression Omnibus under the accession number GSE64666. A complete list of IRF8 depended differentially expressed genes is provided in Supplementary Table 2 . GO analyses were performed using Database for Annotation, Visualization and Integrated Discovery (DAVID; http://david.abcc.ncifcrf.gov/ ) [47] . Immunofluorescence staining and flow cytometry analysis MΦs grown on coverslips were stimulated with required treatment as above. Some cells were treated with 200 nM bafilomycin A1 (Invivogen, cat. no. tlrl-baf) for 2 h, fixed with 4% paraformaldehyde, permeabilized with 0.1% Triton-X-100 for 5 min and blocked by 5% bovine serum albumin with 0.1% Tween 20. Cells were incubated for 5 h with antibody against LC3 (MBL, cat. no. M152-3) or LAMP2 (ProSci, cat. no. 3627), SQSTM1 (MBL, cat. no. PM045), Ubiquitin (Santacruz, cat. no. sc8017) or Listeria (Abcam, cat. no. ab35132) diluted at 1:1,000 followed by 1 h incubation with goat Alexa-488/Alexa-592 anti-rabbit or anti-mouse antibody (Molecular Probes). Cells were counterstained with DAPI for DNA. To detect autophagic vacuoles, mitochondria and lysosomes, cells were incubated with 10 μM Monodansylcadaverine (Sigma 30432), 50 nM MitoTracker red (MT, Invitrogen M22426) or 50 nM LysoTracker-Red (Invitrogen L7528). Stained cells were viewed on a confocal microscope (Leica, SP2) with a × 63 oil immersion objective. Membrane-bound LC3 was detected by the flow cytometry method as described [37] . In brief, the cells were washed with PBS containing 0.05% saponin and incubated with mouse anti-LC3 and then with PE-conjugated goat anti-mouse antibody (Biolegend, cat. no. 405307). Data were analysed using the FlowJo software. Electron microscopy MΦs were fixed in 0.1-M sodium cacodylate buffer pH 7.3 containing 2% paraformaldehyde, 2.5% glutaraldehyde (EMS, 15949) and post fixed with 2% osmium tetroxide in 0.1-M sodium cacodylate buffer and processed as described [35] . Samples were sectioned on a Leica Ultracut UC6 ultramicrotome. Thin sections (70 nm) were post stained with 3% uranyl acetate and Reynolds lead citrate and examined on FEI Tecnai Spirit G2 TEM. Digital images were captured on an FEI Eagle camera. Samples were processed for TEM by the Cell Imaging Facility at Northwestern University Feinberg School of Medicine. Retroviral transduction The assay was performed as described [18] , [20] , [29] . Relevant details are provided in the figure legends. For retroviral transduction, HEK293T retroviral packaging cells were transiently transfected with pMSCV retroviral vectors with WT Irf8 or Irf8K79E using Lipofectamine 2000 according to the manufacturer’s protocol. Retroviral supernatants were collected at 48 h. MФs were transduced by spinoculation (3,000 r.p.m., 33 °C, 1 h) with the retroviral supernatant supplemented with 4 μg ml −1 polybrene. Transduced cells were selected with 2 μg ml −1 puromycin 48 h post spinoculation. Quantitative RT–PCR The assay was performed as described [18] , [20] , [29] . In brief, total RNA was extracted using Trizol (Invitrogen). Complementary DNA was prepared from 1 μg of RNA with Superscript II RT (Invitrogen) and random hexamer primers (Promega). PCR was carried out by ABI 7500 (Applied Biosystems) using a standard protocol for appropriate cycles. Primers used for PCR are listed in Supplementary Table 3 . Transcript levels were normalized by glyceraldehyde-3-phosphate dehydrogenase ( Gapdh ) and fold changes were calculated by the C t method. Immunoblot assay Cell lysates and prestained molecular weight markers were subjected to SDS–polyacrylamide gel electrophoresis and transferred to a nitrocellulose membrane. The membranes were blocked with 5% non-fat milk in TBST (Triton-X-100 containing Tris-buffered saline), incubated with various antibodies (1:3,000) for 1–2 h, washed with TBST, and stained with anti-rabbit or anti-mouse IgG conjugated to peroxidase (1:5,000). Immunoreactivity was visualized by enhanced chemiluminescence (ECL kit, Thermo Fisher Scientific). Full immunoblots with indicated areas of selection are provided in Supplementary Fig. 12 . Chromatin immunoprecipitation assay ChIP assays were performed as previously described [18] , [20] , [29] . In brief, 2.5–10 × 10 6 MФs were crosslinked with 0.75% formaldehyde and quenched in 0.125 M glycine. Cell lysates were sonicated and immunoprecipitated with 0.5 μg of rabbit IgG antibody (Sigma) or anti-IRF8 antibody (affinity purified) [20] . The immunoprecipitated DNA was eluted and amplified by real-time PCR using an ABI 7500 (Applied Biosystems). Values were normalized to corresponding input control and expressed as fold enrichment. Primers used for PCR are listed in Supplementary Table 3 . Statistical analysis Student’s t -test was used as statistical analysis by using Microsoft Excel. How to cite this article: Gupta, M. et al. IRF8 directs stress-induced autophagy in macrophages and promotes clearance of Listeria monocytogenes . Nat. Commun. 6:6379 doi: 10.1038/ncomms7379 (2015).